Direct imaging of light-element impurities in graphene reveals
triple-coordinated oxygen Along with hydrogen, carbon, nitrogen and oxygen are the arguably most
important elements for organic chemistry. Due to their rich variety of possible
bonding configurations, they can form a staggering number of compounds. Here, we
present a detailed analysis of nitrogen and oxygen bonding configurations in a
defective carbon (graphene) lattice. Using aberration-corrected scanning
transmission electron microscopy and single-atom electron energy loss spectroscopy,
we directly imaged oxygen atoms in graphene oxide, as well as nitrogen atoms
implanted into graphene. The collected data allows us to compare nitrogen and oxygen
bonding configurations, showing clear differences between the two elements. As
expected, nitrogen forms either two or three bonds with neighboring carbon atoms,
with three bonds being the preferred configuration. Oxygen, by contrast, tends to
bind with only two carbon atoms. Remarkably, however, triple-coordinated oxygen with
three carbon neighbors is also observed, a configuration that is exceedingly rare in
organic compounds. Recent advances in transmission electron microscopy, in particular
aberration correction, have enabled the study of low-dimensional materials at low
electron energies with atomic resolution. In scanning transmission electron
microscopy (STEM) [1] , the contrast mechanism behind annular dark field
images allows the identification of light elements (e.g. B, C, N, O) despite their
very similar atomic number [2] . In aberration-corrected high-resolution
transmission electron microscopy (HRTEM), however, these elements have an
almost-identical contrast and their discrimination becomes difficult in particular
when they are incorporated into irregular structures such as
defects [3] , [4] . Atomic resolution images have revealed the bonding
configurations of several types of impurities in light-element samples. For example,
nitrogen dopants in graphene and carbon nanotubes have been revealed in several
studies [5] , [6] , [7] , [8] , [9] , boron dopants have been identified in
graphene by STEM [8] , and carbon and oxygen impurities have been
revealed in monolayer hexagonal boron nitride [2] . Oxygen impurities in
graphene are of high relevance due to their importance for the processing of
graphene oxide (GO), and are likely to play a role, e.g. in the degradation of
graphene in oxygen or in air at high temperatures. Despite efforts to quantify the
functional groups in GO [10] , [11] , [12] , [13] , [14] , [15] , the nature of oxygen binding to graphene is
still not well understood. Although few HRTEM studies have revealed disorder and
defects in graphene oxide [16] , [17] , [18] , [19] , a direct visualization of oxygen atoms that
includes their unambiguous chemical identification (e.g., via contrast in STEM or
via electron energy loss spectroscopy, EELS) along with their bonding with a carbon
matrix has not been achieved yet. Here, we study a large number of oxygen impurities in samples of
graphene oxide. The oxygen atoms are identified by their contrast in medium-angle
annular dark field STEM images [2] , and in several cases also by EELS. For
comparison, we also prepared a graphene sample with nitrogen impurities by
low-energy plasma and ion treatment (see the “Methods” section). In contrast to an
earlier study [8] , our samples are transferred under vacuum from
implantation to STEM imaging, which prevents configurations with open bonds from
being saturated with contamination. Our data set is large enough to carry out a
statistical analysis of the different bonding configurations for oxygen and
nitrogen. Moreover, we describe the dynamics of reduction observed under the
electron beam for the case of oxygen. Configurations Before discussing the observed atomic configurations, it must be
pointed out that initial changes occur in the structure of graphene oxide
already at relatively low doses, which makes it challenging if not impossible to
capture the pristine structure in atomic resolution TEM or STEM images. In
agreement with earlier findings [20] , we observed changes in the EELS signal
at doses between 10 3 and
10 6 e − Å −2 (Fig. 1a–d ). We assume that
functional groups which are attached to the basal plane, edges, or defects of
graphene via relatively weak bonds (such as hydroxyl, carboxyl, epoxide, or
ketone groups) are destroyed at these doses before an image could be obtained. Nevertheless, what remains after initial electron irradiation is a defective
graphene sample, where numerous oxygen impurities are incorporated into a
carbonaceous host structure. These structures, which are stable enough for STEM
imaging and in some cases EELS, reveal a variety of bonding configurations for
oxygen in an sp 2 -bonded carbon system. Fig. 1 Reduction of GO under the beam. Lower magnification
(lattice resolution) STEM images: a initial and b after ~50 scans. Adsorbates shrink under observation, and the
clean lattice area increases. The insets show a model with and
without functional groups attached to the graphene sheet
(reduced GO). The upper left section of the image contains the
supporting carbon film. c EEL
spectra after different electron doses showing the loss of the
oxygen K -edge. d EEL intensity of the oxygen K -edge as a function of
electron dose. e High
magnification double-Gaussian filtered image where the graphene
lattice with defects and impurities is resolved. The bright
atoms (red dashed circles) can be identified as oxygen. The atom
in the blue dashed circle is at the edge of the intensity
distribution and might be either nitrogen or oxygen. f Histogram of the ADF intensities of
carbon (gray) and oxygen atoms (red). g Magnified histogram of panel f . Insets in a , b are
reprinted from ref. [10] with permission. Scale
bars are 2 nm Full size image A high-magnification image where the defective carbon honeycomb
lattice can be resolved is presented in Fig. 1 e. While the regular graphene lattice dominates the area of
the sample, a remarkably high density of defects with brighter impurity atoms
can be identified. By analyzing the intensities [2] , most of these atoms can
be assigned as oxygen. 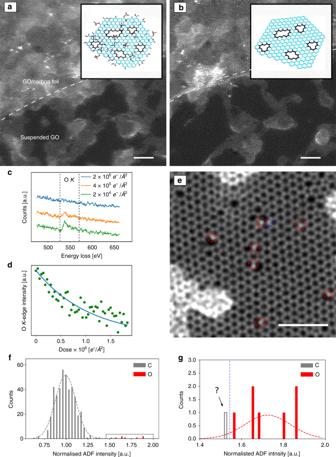Fig. 1 Reduction of GO under the beam. Lower magnification
(lattice resolution) STEM images:ainitial andbafter ~50 scans. Adsorbates shrink under observation, and the
clean lattice area increases. The insets show a model with and
without functional groups attached to the graphene sheet
(reduced GO). The upper left section of the image contains the
supporting carbon film.cEEL
spectra after different electron doses showing the loss of the
oxygenK-edge.dEEL intensity of the oxygenK-edge as a function of
electron dose.eHigh
magnification double-Gaussian filtered image where the graphene
lattice with defects and impurities is resolved. The bright
atoms (red dashed circles) can be identified as oxygen. The atom
in the blue dashed circle is at the edge of the intensity
distribution and might be either nitrogen or oxygen.fHistogram of the ADF intensities of
carbon (gray) and oxygen atoms (red).gMagnified histogram of panelf. Insets ina,bare
reprinted from ref.10with permission. Scale
bars are 2 nm Figure 1f, g show
the histogram of the intensities. We further confirmed the identity for some of
the impurities by EELS (which in turn validates the intensity analysis). Due to
a lower dose than that used in ref. [2] necessitated by the sample stability, a
small fraction of the impurities cannot be uniquely assigned, e.g. where the
tails between the nitrogen and oxygen intensity distribution overlap in the
histogram (Fig. 1g ). For example, the
atom in Fig. 1c marked by the blue
circle could—based on the intensity alone—be either nitrogen or oxygen. However,
since the EELS signal of the GO samples shows no indication of nitrogen, we
assume the impurity atom to be oxygen in such cases. For the N-doped graphene, we classify the configurations in
agreement with earlier literature into graphitic (substitution with three N–C
bonds), pyridinic (two N–C bonds in a hexagon) and pyrrolic (two N–C bonds in a
pentagon) configurations. Different oxygen and nitrogen configurations are shown
in Fig. 2 . Fig. 2 STEM images of different configurations of oxygen and
nitrogen atoms in graphene. a Oxygen pair. b Graphitic
substitution by oxygen. c Oxygen atoms within vacancies. d Nitrogen-doped graphene configurations. e Distribution of the
different configurations in GO (red) and N-doped graphene
(blue). f Distribution of
double-coordinated and triple-coordinated heteroatoms in GO
(red) and N-doped graphene (blue). N shows the total number of heteroatoms of each
sample (note that some configurations contain multiple
heteroatoms). Scale bars are 0.5 nm Full size image For the oxygen impurities, the conventional classification into
different types of functional groups is not useful for describing the observed
structures. Instead, we classify the oxygen configurations into three frequently
observed types. The first, and surprisingly frequently observed, configuration
consists of two oxygen atoms substituting two neighboring carbon atoms. An
example of a STEM image of this configuration is shown in Fig. 2a . Graphitic substitutions are our second type
of configuration (Fig. 2b ). This is the
only configuration in which oxygen binds with three carbon neighbors, similar to
the oxygen impurities imaged in hexagonal boron nitride [2] . Our third class of
configurations are oxygen atoms next to vacancies. Interestingly, they form
defect reconstructions that are very similar to those in graphene without
heteroatoms, except that one or two carbon atoms at the edge of a vacancy are
replaced by oxygen. We label these defects in accordance with the carbon-only
structures. In a 5–9 monovacancy (MV) [21] , for example, a single oxygen replaces
the carbon atom with only two bonds (Fig. 2c , first column) while the structure undergoes a distortion
that looks like the Jahn–Teller distortion of a carbon-only vacancy. If two
oxygen atoms are present, however, both remain two-coordinated and the bond at
the pentagon remains open leading to a symmetric MV configuration
(Fig. 2c , second column). Another
prominent example is the divacancy (DV) [22] , where two oxygen atoms
can sit in the same pentagon of a 5-8-5 DV (third column of Fig. 2c ). Also here, the two oxygen atoms do not form
a bond and have a larger projected distance than the corresponding carbon atoms
at the opposite pentagon. The 555–777 DV (fourth column) shows an interesting
behavior when one carbon is replaced by an oxygen atom: Here, the oxygen only
binds with two carbon atoms, breaking the three-fold symmetry. In a
configuration where three carbon atoms are missing (last column of
Fig. 2c ), the oxygen atom binds with
two carbon atoms building a “bridge”. This appears very similar to a graphene
trivacancy (TV). All of these configurations, except for the graphitic type,
form an ether-like bond, i.e. an oxygen binding to two different carbon
atoms. A statistical analysis of the distribution of the configurations
reveals that the oxygen pair is the most prominent one (Fig. 2e ), whereas the graphitic substitution is the
least frequent. In contrast, in our N-doped graphene sample, the pyrrolic
configuration was the most favored one followed by the graphitic substitution. The occurrence of the pyridinic configuration is low in our case. It can be
increased by ozone treatment during sample preparation [23] , which we have not
done. The difference of the bonding configurations of N and O in graphene can be
highlighted by the distribution of their coordination numbers (Fig. 2f ). The statistical analysis of our atomic
resolution images directly confirms that oxygen prefers two bonds while nitrogen
prefers three bonds. This is in agreement with the different electronic
configuration of these elements, and hence different preferences for forming
chemical bonds with carbon. To analyze their structural properties, we performed density
functional theory (DFT) calculations for each configuration. The obtained
relaxed models are shown below the STEM images in Fig. 2 . In some cases, we find clear differences in the structural
relaxation for oxygen in comparison to nitrogen. For example, the relaxed
structure of the 555–777 DV (Fig. 2c ,
fourth column) shows a large projected distance of the oxygen atom to one of its
three neighbors, breaking the three-fold symmetry of this configuration. Clearly, the oxygen in this case binds only with two carbon atoms. However, a
nitrogen atom in the same position results in a highly symmetric configuration
with three neighbors close to the impurity (Supplementary Fig. 2 ). For the double-oxygen site
(Fig. 2a ), the two oxygen atoms do
not bind but stick out of the graphene plane in opposite directions, with a
projected distance that is significantly larger than the carbon–carbon bond in
graphene. This is not the case for a simulated double-nitrogen structure
(see Supplementary Discussion ). All other considered configurations have very similar structural properties for
both nitrogen and oxygen impurities, except for small out-of-plane
displacements. The energies of the relaxed configurations with the heteroatoms
incorporated in the lattice ( E in ) for both, nitrogen and oxygen, were
also obtained by DFT. We calculated the sum of the energies ( E out + E isolated ) when the
heteroatoms are released from the lattice (after relaxation) and the isolated
atoms (half of N 2 or O 2 ). The
difference E in − ( E out + E isolated ) is referred as binding energy
and is lower (meaning higher stability) for all N configurations. This is in
agreement with the observed higher stability of N dopants in graphene. 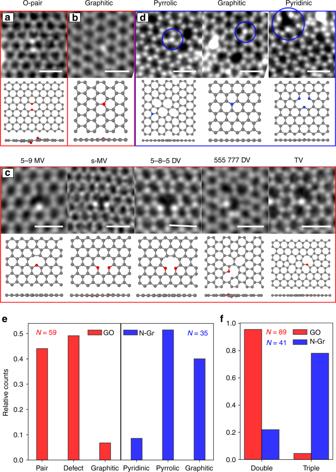Fig. 2 STEM images of different configurations of oxygen and
nitrogen atoms in graphene.aOxygen pair.bGraphitic
substitution by oxygen.cOxygen atoms within vacancies.dNitrogen-doped graphene configurations.eDistribution of the
different configurations in GO (red) and N-doped graphene
(blue).fDistribution of
double-coordinated and triple-coordinated heteroatoms in GO
(red) and N-doped graphene (blue).Nshows the total number of heteroatoms of each
sample (note that some configurations contain multiple
heteroatoms). Scale bars are 0.5 nm All
calculated energies are listed in Supplementary Table 2 . The binding energies are negative in all
cases, which means that the structures are stable with respect to forming a
carbon-only vacancy plus isolated O or N. Dynamics The oxygen substitutions are sputtered after a dose with a
geometrical mean of
5 × 10 5 e − Å −2 and replaced by a carbon atom, whereas nitrogen substitutions can withstand
orders of magnitude higher doses [24] (cf. Fig. 3a–c ). 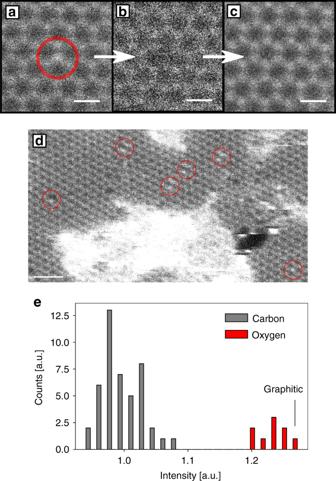Fig. 3 Graphitic oxygen substitution.aUnprocessed STEM image of a graphitic oxygen
substitution in graphene.bOxygen atom is sputtered after four frames, leaving a vacancy.cPristine graphene lattice
after the vacancy gets refilled by a carbon atom.dLow-magnification image of the GO
sample, where multiple pair configurations and a graphitic
substitution is present.eHistogram of intensity distribution of atoms in paneld. Scale bars in panela–cand in paneldare 0.25 and
1 nm, respectively To understand this difference, we performed DFT-based
molecular dynamics calculations (see the “Methods” section). The threshold
energy for removing an oxygen atom from the lattice is 10.3 eV, and the
threshold for removing the neighboring carbon is 15.0 eV. This energy is almost
2/3 of the calculated 22.0 eV threshold kinetic energy for a carbon in pristine
graphene and also significantly lower than for nitrogen in graphene
(19.09 eV) [25] . Indeed, graphitic nitrogen in graphene was
found to be extremely stable under 60 or 80 kV electron irradiation, such that
the atomic structure of the dopant site is more likely to be changed by
displacing a neighboring carbon atom before the dopant atom itself is sputtered
under electron irradiation [25] . Hence, the observed clear difference in
the stability under the beam between graphitic oxygen and nitrogen impurities is
in agreement with the calculations. We further performed intensity analysis of
another STEM image, where multiple oxygen pair configurations, as well as a
graphitic configuration are present (see Fig. 3d ). The histogram of the atom intensities (Fig. 3e ) shows that the intensity of the graphitic
configuration is clearly within the distribution of oxygen. Fig. 3 Graphitic oxygen substitution. a Unprocessed STEM image of a graphitic oxygen
substitution in graphene. b Oxygen atom is sputtered after four frames, leaving a vacancy. c Pristine graphene lattice
after the vacancy gets refilled by a carbon atom. d Low-magnification image of the GO
sample, where multiple pair configurations and a graphitic
substitution is present. e Histogram of intensity distribution of atoms in panel d . Scale bars in panel a – c and in panel d are 0.25 and
1 nm, respectively Full size image As mentioned above, we often observed the neighboring double-oxygen
configuration as shown in Fig. 4a . Calculations [26] and experiments [27] show that directly
neighboring nitrogen atoms are energetically unfavorable, while our experiments
indicate that in the case of oxygen such a configuration is stable. Interesting
dynamics can be observed when one oxygen atom is sputtered and a MV
configuration with a single oxygen atom is left behind (Fig. 4b, c ): During imaging, the oxygen atom jumps
frequently to the opposite vacancy site. Similar dynamics were reported in a
N-doped sample [5] . The number of images between such events
spans the range from 1 to 15 with a dose of ca. 6 × 10 5 e − Å −2 per image. After a long electron exposure, the second O atom can be removed,
leaving behind a DV (Fig. 4d ), which is
also highly dynamic [22] . A video of this process is shown in
the Supplementary
Discussion . Fig. 4 In situ oxygen reduction and dynamics in GO. a STEM image of the oxygen pair
configuration. b , c One oxygen is released after
several scans, creating a vacancy beside the oxygen atom. The
oxygen atom jumps frequently to the opposite equivalent site. d Second oxygen is knocked
out after several scans creating a divacancy. e EEL spectrum of a double-O
configuration, which converted into single-O during spectrum
acquisition (total dose: ca. 2 × 10 10 e − Å −1 ). f Reduction process of
oxygen. g Rotation of the 5-8-5
DV with two oxygen atoms. Scale bar is 0.5 nm Full size image Another example of dynamics is shown in Fig. 4f . In this case, two oxygen atoms were found in
a MV. After a few images, one carbon is sputtered and a 5-8-5 DV with two oxygen
atoms forms (cf. Fig. 2c , middle
column). Then, after a few scans, one oxygen is removed and after
some intermediate (not clearly observed) steps, a structure with two defects, a
MV and a 555–777 DV, is formed. These observations indicate that, similar to
all-carbon defects in graphene, also carbon–oxygen configurations can undergo
beam-induced bond rotations and thereby migrate in the
lattice [22] . 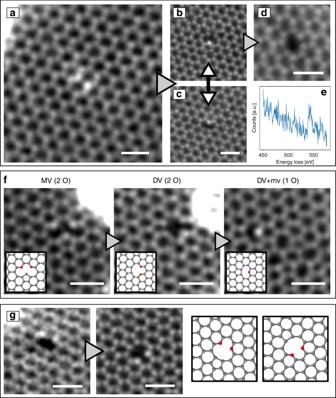Fig. 4 In situ oxygen reduction and dynamics in GO.aSTEM image of the oxygen pair
configuration.b,cOne oxygen is released after
several scans, creating a vacancy beside the oxygen atom. The
oxygen atom jumps frequently to the opposite equivalent site.dSecond oxygen is knocked
out after several scans creating a divacancy.eEEL spectrum of a double-O
configuration, which converted into single-O during spectrum
acquisition (total dose: ca.
2 × 1010e−Å−1).fReduction process of
oxygen.gRotation of the 5-8-5
DV with two oxygen atoms. Scale bar is 0.5 nm Figure 4g shows the 5-8-5 DV in two distinct, but equivalent
states. Oxygen with three carbon neighbors appears as a surprise, because it
seems to contradict the textbook concept of oxygen forming two bonds (or one double
bond), while nitrogen forms three, and carbon up to four covalent bonds. Within the
known organic compounds, trivalent oxygen only appears in a charged state, referred
to as oxonium, and is difficult to stabilize in extended
compounds [28] . Here, the oxygen with three carbon neighbors is
found in an extended organic matrix, and the fact that it survives sufficient dose
of high-energy electrons for recording several high-resolution images means that it
must have a remarkable stability. With respect to the structure of GO, our results indicate that oxygen
atoms incorporated into the graphene lattice or integrated into small defects within
in the graphene plane could play an important role among the structural
configurations in GO or reduced GO. In particular, the high stability of these
configurations means that they would be difficult to remove, e.g. by thermal
annealing. Indeed, several of our configurations appear to have been predicted by
simulations of oxidation and annealing of graphene (Fig. 2 of
ref. [29] ), and formed under simulated annealing
conditions where most functional groups attached to the basal plane were
removed. In conclusion, we have shown a large variety of bonding configurations
of nitrogen and oxygen atoms in a carbon matrix via atomic resolution imaging. For
the first time, individual oxygen impurities were clearly identified, and a
statistical analysis for both oxygen-containing and nitrogen-containing defects was
presented. By and large, the preference of nitrogen for three bonds, versus the
preference of oxygen for two bonds, is confirmed. An oxygen pair configuration is
revealed to be a very frequent configuration in GO, followed by different types of
double-coordinated oxygen atoms at the edges of vacancies. As a remarkable minority,
symmetric, graphitic substitutions of oxygen binding to three carbon neighbors in
graphene were found. Further, we presented electron-beam-induced reduction dynamics. Overall, we find that the structural features of the defects are similar for
all-carbon defects compared to nitrogen-containing or oxygen-containing defects in
the same configuration, while differences in the bond lengths or stability are
nevertheless detectable. Sample preparation GO is usually prepared from graphite oxide [30] , [31] , [32] by mixing graphite powder into an acid
solution, which leads to oxidation. In an improved method, the temperature
during oxidation is kept low in order to suppress the extensive formation of
CO 2 , which therefore improves the quality of the
sample [33] . Water dispersion of graphene oxide was
received from the company Danubia NanoTech, Ltd. The oxidation method of
graphitic powder and subsequent exfoliation were developed with a goal to
preserve the long-range structural order in the graphene oxide flakes exfoliated
down to the single-atom thickness. Water dispersion of GO was significantly
diluted (ca. 1:100). A TEM grid was then vertically dipped into the dispersion
for one minute and dried in air afterwards. Nitrogen-doped samples prepared for comparison were made by
irradiating graphene on TEM grids (obtained from Graphenea) with 50 eV nitrogen
ions [26] . The plasma irradiation was carried out in a
target chamber that is directly connected to the Nion microscope via a UHV
transfer system [34] . The sample was irradiated for 16 min at a
pressure of ca. 3 × 10 −6 mbar, resulting in a total
ion dose of 4 ions nm −2 . During irradiation, the
sample was heated with a laser (270 mW) in order to reduce contamination. The
irradiation treatment in the vacuum system is very similar to the preparation in
ref. [34] except that we used nitrogen instead of
argon. As a result, we find numerous defects where open bonds can still be
observed, e.g., the pyridinic nitrogen configuration (which would likely be
covered with contamination if the sample were transferred through air) without
post-annealing the sample [5] . Electron microscopy STEM experiments were conducted using a Nion UltraSTEM100, operated
at 60 kV. Typically, our atomic-resolution images were recorded with 512 × 512
pixels for a field of view of 6–8 nm and dwell time of 16 μm per pixel using the
medium angle annular dark field (MAADF) detector with an angular range of
60–200 mrad. The probe current was ~20 pA and the beam (semi-)convergence angle
was 30 mrad. Where appropriate if the structure did not change, a few (2–5)
experimental images were averaged in order to increase the signal-to-noise
ratio. Intensity analysis The histograms show integrated atom intensities of the
double-Gaussian processed STEM images. The parameters for the filter are similar
as in ref. [2] so that the maximum of the double-Gaussian
function is between the first two orders of the graphene peaks in the reciprocal
space. The width of the Gaussian fit of the carbon peak is assumed to be the
same as for the intensity distribution of the other elements. Density functional theory We used DFT as implemented in the Vienna ab initio simulation
package (VASP) [35] within the generalized gradient
approximation of Perdew, Burke, and Ernzernhof (PBE) for exchange and
correlation [36] . Projector-augmented wave (PAW)
potentials [37] were used to describe the core electrons. The kinetic energy cutoff was 700 eV. In case of oxygen impurities, a
spin-polarized density-functional method was used. Depending on the defect size
and number of impurity atoms, different supercells were selected for modeling. The smallest one was a 5 × 5 × 1 supercell with 50 atoms for the nitrogen
graphitic impurity,whereas a 8 × 8 × 1 supercell containing 128 atoms was used
for the TV defect. For all defect structures, a Γ-centered k -point sampling was used for the Brillouin-zone
integration. The k -point meshes were selected
to correspond to 36 × 36 × 1 points for the unit cell of graphene. The
structures were fully optimized using the damped molecular dynamics method until
the residual forces were smaller than 0.005 eV Å −1 . Due to the size of the defects and existing impurities, special care was devoted
to minimize the external pressure or strain on the supercells calculated from
traces of the stress tensor. The total energies were calculated based on
supercell sizes with minimum external pressure. To calculate the displacement threshold energy, we carred out
DFT/MD calculations at 300 K using the Langvin NVT thermostat. In these
simulations, appropriate velocity is given to the oxygen atom and the simulation
is run with a 0.5 fs time step for 100 fs. The calculation is then repeated for
the neighboring carbon atom.